MXene molecular sieving membranes for highly efficient gas separation 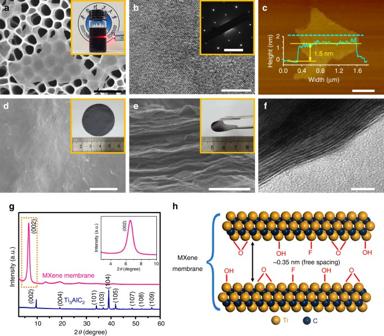Fig. 1 Morphology and structure of exfoliated MXene (Ti3C2TX) nanosheets and stacked MXene membrane.aSEM image of the delaminated MXene nanosheets on porous anodic aluminum oxide (AAO) (scale bar, 1 μm). Inset is the Tyndall scattering effect in MXene colloidal solution in water.bHRTEM image of the MXene nanosheet with SAED pattern in the inset (scale bar, 5 nm, insetb, 5 nm−1).cAFM image of the MXene nanosheet on cleaved mica. The height profile of the nanosheet corresponds to the blue dashed line (scale bar, 500 nm). Note that the adsorbed molecules, such as H2O, also contribute the detected thickness of 1.5 nm.dSEM image of the MXene membrane surface (scale bar, 500 nm). Inset is a photograph of a MXene membrane.eCross-sectional SEM image of the MXene membrane (scale bar, 1 μm). Inset is a tweezer bent membrane.fCross-sectional TEM image of the MXene membrane with 2D channels (scale bar, 10 nm).gXRD patterns of the MAX (Ti3AlC2) powder and MXene (Ti3C2TX) membrane with inset of the magnified XRD pattern at low Bragg angles.hIllustration of the spacing between the neighboring MXene nanosheets in the membrane Molecular sieving membranes with sufficient and uniform nanochannels that break the permeability-selectivity trade-off are desirable for energy-efficient gas separation, and the arising two-dimensional (2D) materials provide new routes for membrane development. However, for 2D lamellar membranes, disordered interlayer nanochannels for mass transport are usually formed between randomly stacked neighboring nanosheets, which is obstructive for highly efficient separation. Therefore, manufacturing lamellar membranes with highly ordered nanochannel structures for fast and precise molecular sieving is still challenging. Here, we report on lamellar stacked MXene membranes with aligned and regular subnanometer channels, taking advantage of the abundant surface-terminating groups on the MXene nanosheets, which exhibit excellent gas separation performance with H 2 permeability >2200 Barrer and H 2 /CO 2 selectivity >160, superior to the state-of-the-art membranes. The results of molecular dynamics simulations quantitatively support the experiments, confirming the subnanometer interlayer spacing between the neighboring MXene nanosheets as molecular sieving channels for gas separation. Gas separation with membrane technology is attractive because of its high efficiency, low energy consumption, and simple operation [1] , [2] , [3] . Membranes with high permeability and high selectivity are urgently required [3] . The recent use of two-dimensional (2D) materials [4] , [5] , such as graphene and graphene oxide (GO) [6] , [7] , [8] , [9] , [10] , [11] , [12] , [13] , zeolite or metal–organic framework (MOF) nanosheets [14] , [15] , [16] , has led to innovative membrane designs. Previous studies have shown that MOF nanosheets are promising for membrane assembly [15] , [16] and a pioneering breakthrough work on zeolite nanosheets based membrane was also conducted by Tsapatsis [14] , [17] , [18] , [19] , where the molecules were mainly transported through the intrinsic pores in the 2D nanosheets. But the types of zeolite or MOFs that can be easily exfoliated are rather limited due to the structural deterioration in exfoliation process [15] , [16] . Similarly, the monolayer graphene with artificial sub-nanopores created by selective etching or ion bombardment is emerged as selective membrane for gas separation or ion sieving [20] , [21] , [22] . However, it is difficult to fabricate the graphene sheets with controllable and uniform pores due to the stochastic nature, which limits the industrial applications. In contrast to the membranes with intrinsic or artificial pores on the nanosheets as the main molecular sieving channels, another kind of 2D laminar membrane has attracted increasing attention due to its simple preparation and easy to large-scale fabrication, in which the molecules are transported and sieved through the interlayer nanochannels between the neighboring nanosheets [6] , [7] , [8] , [23] . Therefore, for the latter 2D laminar membranes, the stacking structure of the nanosheets strongly affects the separation performance [6] , [7] , [8] . For instance, a GO membrane with randomly stacked structure exhibited only Knudsen diffusion during gas separation, while a membrane with an ordered structure exhibited molecular sieving with a greatly increased gas separation factor [6] . Moreover, many other well-ordered GO laminates exhibited enhanced gas or water separation performance in terms of their selectivity and permeability compared to the disordered ones [7] , [8] . However, since the oxygen-containing functional groups that decorate the defects in GO sheets are difficult to control, random laminar structures are easily formed when such sheets are stacked into membranes [7] , [8] . Another young family of 2D materials named “MXenes” with the formula of M n +1 X n T X , are usually produced by selectively etching the A-group (mainly group IIIA or IVA elements) layers from M n +1 AX n phases ( n = 1, 2, or 3), where M is an early transition metal and X is carbon and/or nitrogen. More importantly, abundant of surface-terminating groups (T X : = O, –OH and –F) are formed evenly on the entire surface of the nanosheets during the etching and delaminating processes [24] , [25] , [26] , [27] , [28] , [29] , [30] , [31] . Interestingly, the variety of T X species can create open narrow nanochannels between the neighboring nanosheets in stacked MXene laminates, making MXene a promising material to assemble highly efficient membranes [27] . Here, exfoliated MXene nanosheets were used as building blocks to construct 2D laminated membranes for selective gas separation for the first time, as demonstrated using a model system of H 2 and CO 2 . The MXene membranes exhibit excellent performance in terms of the hydrogen permeability and H 2 /CO 2 selectivity, transcending the state-of-the-art membranes. Such high-permeability hydrogen-selective membranes are desired in many fields, such as hydrogen production and carbon dioxide capture. Preparation of MXene nanosheets The most common MXene, Ti 3 C 2 T X , is obtained after selectively etching Al from the corresponding MAX (Ti 3 AlC 2 ) phase using hydrochloric acid and lithium fluoride [24] , [25] , [26] , [29] , the structures are displayed in Supplementary Fig. 1 and explained in Supplementary Note 1 . The Tyndall scattering effect in the as-prepared MXene colloidal suspension is clearly observed (Fig. 1a , inset, Supplementary Fig. 2 , and Supplementary Note 2 ). The scanning electron microscopy (SEM) and transmission electron microscopy (TEM) images (Fig. 1a and Supplementary Fig. 3 ) show that the exfoliated MXene nanosheets are very thin and nearly transparent to the electron beams. 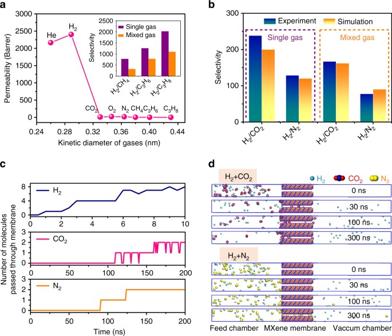Fig. 2 MD simulations of the gas permeation through the MXene membrane compared with the experimental results.aSingle-gas permeabilities through a 2-μm-thick MXene membrane as a function of the gas kinetic diameter at 25 °C and 1 bar. Inset shows the selectivity of H2relative to the other gases in both the single-gas and equimolar mixed-gas permeation studies.bComparison of the experimental and MD simulated selectivities of H2/CO2and H2/N2in both the single-gas and mixed-gas permeations.cThe number of gas molecules that passed through the MXene membrane in MD simulation as a function of simulation time for single-gas permeation. For H2, only the first 10 ns of the simulation are shown because of its fast permeation. By contrast, only two molecules pass through the MXene membrane during the 200-ns-long simulation for CO2or N2. The CO2curve fluctuates because of CO2adsorption–desorption on the MXene membrane.dSimulation snapshots at 0, 30, 100, and 300 ns for two sets of mixed-gas permeation systems: (H2+ CO2) and (H2+ N2). Note that H2was modeled by united-atom force field. The MXene membrane was composed of two nanosheets with a free spacing of 0.35 nm located in the middle of the simulation system. In the beginning (t= 0 ns), 30 H2and 30 CO2(or N2) molecules were present in the feed chamber, which permeated through the MXene membrane to the evacuated permeate chamber. The details can be found in section of “Methods” 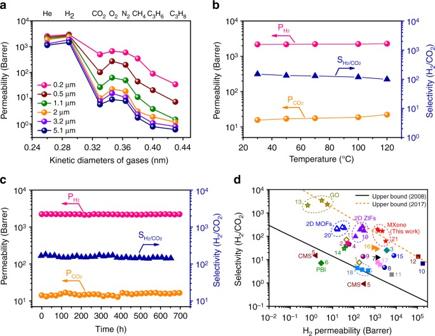Fig. 3 Gas separation performance of the MXene membrane.aSingle-gas permeabilities through the MXene membranes with different thicknesses at 25 °C and 1 bar.bH2/CO2separation performance of a 2-μm-thick MXene membrane as a function of temperature in the equimolar mixed-gas permeation.cLong-term separation of equimolar H2/CO2mixture through a 2-μm-thick MXene membrane at 25 °C and 1 bar.dH2/CO2separation performance of the MXene membrane compared with state-of-the-art gas separation membranes. The black line indicates the Robeson 2008 upper bound of polymeric membranes for H2/CO2separation58, and the orange dashed line represents the 2017 upper bound of the best current membranes for H2/CO2separation. Information on the data points is given in Supplementary Table9 High-resolution TEM (HRTEM) image and selected-area electron diffraction (SAED) patterns (Fig. 1b and Supplementary Figs. 4 and 5 ) indicate the hexagonal structure of the basal planes and high crystallinity of the MXene flakes without obvious nanometer-scale defects or carbide amorphization. As indicated from the atomic force microscopy (AFM) measurements (Fig. 1c and Supplementary Fig. 6 ), most of the MXene nanosheets have a uniform thickness of 1.5 nm with a lateral size of 1–2 μm. Considering that the theoretical thickness of a Ti 3 C 2 T X single layer is ~1 nm [29] , [32] , and MXene nanosheets adsorb water and other molecules that also contribute to the total thickness, the 1.5-nm-thick nanosheet should be monolayer Ti 3 C 2 T X [26] , [32] . Fig. 1 Morphology and structure of exfoliated MXene (Ti 3 C 2 T X ) nanosheets and stacked MXene membrane. a SEM image of the delaminated MXene nanosheets on porous anodic aluminum oxide (AAO) (scale bar, 1 μm). Inset is the Tyndall scattering effect in MXene colloidal solution in water. b HRTEM image of the MXene nanosheet with SAED pattern in the inset (scale bar, 5 nm, inset b , 5 nm −1 ). c AFM image of the MXene nanosheet on cleaved mica. The height profile of the nanosheet corresponds to the blue dashed line (scale bar, 500 nm). Note that the adsorbed molecules, such as H 2 O, also contribute the detected thickness of 1.5 nm. d SEM image of the MXene membrane surface (scale bar, 500 nm). Inset is a photograph of a MXene membrane. e Cross-sectional SEM image of the MXene membrane (scale bar, 1 μm). Inset is a tweezer bent membrane. f Cross-sectional TEM image of the MXene membrane with 2D channels (scale bar, 10 nm). g XRD patterns of the MAX (Ti 3 AlC 2 ) powder and MXene (Ti 3 C 2 T X ) membrane with inset of the magnified XRD pattern at low Bragg angles. h Illustration of the spacing between the neighboring MXene nanosheets in the membrane Full size image Preparation of 2D MXene membranes The MXene membranes were fabricated using vacuum-assisted filtration on anodic aluminum oxide (AAO) support (Fig. 1a and Supplementary Fig. 7 ). After detaching the MXene layers from the substrate, free-standing MXene membranes were directly obtained with good flexibility (Fig. 1e and Supplementary Figs. 8 and 9 ). From the top-view SEM and AFM images (Fig. 1d and Supplementary Fig. 10 ), the membrane is determined to be intact, and the terminating groups were also detected on the MXene membrane (see Supplementary Figs. 11 – 17 and Supplementary Tables 1 – 3 for the Fourier transform infrared spectroscopy (FTIR), thermogravimetric analysis (TGA), energy dispersive X-ray spectroscopy (EDX), and X-ray photoelectron spectroscopy (XPS) results). The cross-sectional SEM image and elemental distribution (Fig. 1e and Supplementary Figs. 13 – 15 ) indicate a homogeneous laminar structure throughout the membrane. The cross-sectional TEM images (Fig. 1f and Supplementary Fig. 18 ) reveal well-organized, highly ordered subnanometer channels resulting from the evenly distributed terminating groups on the MXene nanosheet surface [30] , [33] , [34] . The sharp (002) peak with high intensity in the powder X-ray diffraction (XRD, Fig. 1g ) results further confirms the ordered stacking in the MXene membrane. The (002) peak at 2 θ = 6.6° indicates the d -spacing of ~1.35 nm, based on Bragg’s law (Supplementary Fig. 19 , Supplementary Note 3 , and Supplementary Equation ( 2) ). After deducting the monolayer thickness of ~1 nm [29] , [32] , the free spacing between the neighboring MXene nanosheets is estimated to be ~0.35 nm (Fig. 1h ), which could serve as a molecular sieve to separate gases by membrane permeation. Gas separation performance of 2D MXene membranes The MXene membranes were sealed into Wicke–Kallenbach permeation cells to measure the gas separation performance (Supplementary Figs. 20 and 21 ). For our MXene membrane, the permeability of the small gas molecules (2164 Barrer for He and 2402 Barrer for H 2 ) is much higher than that of the gases with bigger kinetic diameters (Fig. 2a and Supplementary Table 4 ), showing a clear cutoff in between. The ideal selectivity (238.4) of the single-gas permeation and the separation factor (166.6) of the mixed-gas permeation of H 2 /CO 2 are much higher than the corresponding Knudsen coefficient (4.7). Obviously, the gas permeation is mainly dominated by the gas kinetic diameter rather than its molecular weight (Fig. 2a and Supplementary Fig. 22 ), known as the molecular sieving (size exclusion) mechanism. Very interestingly, the permeability of CO 2 (10 Barrer) is approximately half of N 2 (19 Barrer), although its kinetic diameter (0.33 nm) is 9% smaller than that of N 2 (0.364 nm). Here, adsorption modifies the molecular sieving process. Because CO 2 has a much larger quadrupole moment than N 2 , it interacts with the MXene membrane stronger (the interaction energy values of MXene with CO 2 and N 2 , as calculated by molecular dynamics (MD) simulations, are −175.1 and −97.5 kJ mol −1 , respectively, see Supplementary Note 4 and 5 ), which considerably suppress the CO 2 diffusion in the MXene subnanometer channels [6] , [7] . The adsorption isotherms of the gases on the MXene membranes at 25 °C also indicate a preferential adsorption of CO 2 compared to N 2 or other gases (Supplementary Fig. 23 ), even though the adsorption capacities of the MXene nanosheets are quite small [15] , [16] , [35] . The adsorbed CO 2 molecules in the subnanochannels can even block the passing molecules and increase the resistance to CO 2 diffusion, while such phenomenon is absent for H 2 , resulting a high separation factor of H 2 /CO 2 . For O 2 , its kinetic diameter (0.346 nm) is just slightly smaller than the interlayer spacing of the MXene membrane (0.35 nm). Although O 2 can pass through the subnanochannels in the membrane, but with a much larger mass transfer resistance due to the confinement of the neighboring MXene nanosheets. That is why the O 2 permeability is significantly lower than that of much smaller molecules, such as He and H 2 . Fig. 2 MD simulations of the gas permeation through the MXene membrane compared with the experimental results. a Single-gas permeabilities through a 2-μm-thick MXene membrane as a function of the gas kinetic diameter at 25 °C and 1 bar. Inset shows the selectivity of H 2 relative to the other gases in both the single-gas and equimolar mixed-gas permeation studies. b Comparison of the experimental and MD simulated selectivities of H 2 /CO 2 and H 2 /N 2 in both the single-gas and mixed-gas permeations. c The number of gas molecules that passed through the MXene membrane in MD simulation as a function of simulation time for single-gas permeation. For H 2 , only the first 10 ns of the simulation are shown because of its fast permeation. By contrast, only two molecules pass through the MXene membrane during the 200-ns-long simulation for CO 2 or N 2 . The CO 2 curve fluctuates because of CO 2 adsorption–desorption on the MXene membrane. d Simulation snapshots at 0, 30, 100, and 300 ns for two sets of mixed-gas permeation systems: (H 2 + CO 2 ) and (H 2 + N 2 ). Note that H 2 was modeled by united-atom force field. The MXene membrane was composed of two nanosheets with a free spacing of 0.35 nm located in the middle of the simulation system. In the beginning ( t = 0 ns), 30 H 2 and 30 CO 2 (or N 2 ) molecules were present in the feed chamber, which permeated through the MXene membrane to the evacuated permeate chamber. The details can be found in section of “Methods” Full size image Gas separation mechanism To elucidate the gas separation mechanism, two sets of atomistic MD simulations (total simulation time >5 μs) were performed to study the gas transport through the MXene membrane, as schematically shown in Supplementary Fig. 24 [16] , [36] . First, the confined diffusion coefficients of He, H 2 , CO 2 , O 2 , N 2 , and CH 4 in two neighboring MXene channels with 0.35 nm free spacing were calculated by MD simulations (Supplementary Fig. 25 and Supplementary Note 4 ) [37] . The simulation yields a diffusivity ratio of 175:238:1.0:4.1:1.4:0.1. Furthermore, hundreds-nanosecond (ns)-long MD simulations were carried out to study the passage of the gas molecules through the MXene membrane [16] , [36] . In simulations of single-gas permeation (Fig. 2b, c , Supplementary Fig. 26 , and Supplementary Note 5 ), the fluxes of H 2 , CO 2 , O 2 , and N 2 transporting from the feed to permeate chamber are 0.75, 0.0038, 0.0071, and 0.0063 molecule ns −1 , respectively (each value are estimated from the average of four 200-ns-long MD simulations, except for the H 2 flux) (Supplementary Table 5 ). The simulated selectivities of H 2 /CO 2 (200) and H 2 /N 2 (120) are comparable to their respective experimental values of 238 and 129 (Fig. 2b ). From the mixed-gas separation simulations (Fig. 2d ), the selectivities of H 2 /CO 2 (162) and H 2 /N 2 (90), averaged from four 300-ns-long MD simulations, are close to the corresponding experimental selectivities of 167 and 78 (Fig. 2b and Supplementary Table 6 ). Both the MD simulations and experiments show that the gas molecules with sizes much smaller than the free spacing between the neighboring nanosheets (e.g., H 2 and He) move through the membrane quickly. By contrast, the gas molecules with sizes larger (or only slightly smaller) than the free spacing (O 2 , N 2 , and CH 4 ) move 100 times slower because of the molecular sieving mechanism, resulting in gas separation selectivity above 100. For the gas molecule with specific adsorptive property, such as CO 2 , its interaction with MXene considerably affects the gas transport rate, which further increases the H 2 /CO 2 selectivity. The quantitative agreement between the MD simulations and experiments indicates that molecular sieving occurs during gas separation through the MXene membrane. Generally, terminations on the surface of a 2D membrane may affect the separation performance in some cases, therefore, another model using –F termination (i.e., Ti 3 C 2 F 2 ) has also been built to investigate the effect of different terminations on the MD simulated gas permeation (Supplementary Table 7 , Supplementary Fig. 27 , and Supplementary Note 6 ). The results show that there is no significant difference between the gas permeation in two simulation systems. Moreover, the gas separation performance of the MXene membranes can be optimized by adjusting the membrane thickness, temperature, feeding H 2 concentration, and feed gas pressure (Fig. 3a, b , Supplementary Figs. 28 – 33 , and Supplementary Note 7 ). The MXene membrane shows stable performance during a 700 h continuous separation of H 2 /CO 2 mixture (Fig. 3c ). No deterioration was observed even when the feed gas contained 3 vol% steam (Supplementary Fig. 34 ). And the MXene membranes also show good reproducibility (Supplementary Table 8 ). Further, the 2-μm-thick MXene membrane also exhibits tensile strength above 50 MPa and Young’s modulus of 3.8 GPa, showing good mechanical properties (Supplementary Fig. 35 and Supplementary Note 8 ). Compared with various previously reported membranes (Fig. 3d , Supplementary Table 9 , and Supplementary Note 9 ), the MXene membrane exhibits both great H 2 permeability (>2200 Barrer) and high H 2 /CO 2 selectivity (>160), which considerably exceeds the latest upper bound of most current membranes. This promising separation performance is attributed to the regular subnanometer channels in the stacked MXene membrane, and the pivotal role of the regular structure in separation have also been further verified using MD simulation (Supplementary Note 6 ). Fig. 3 Gas separation performance of the MXene membrane. a Single-gas permeabilities through the MXene membranes with different thicknesses at 25 °C and 1 bar. b H 2 /CO 2 separation performance of a 2-μm-thick MXene membrane as a function of temperature in the equimolar mixed-gas permeation. c Long-term separation of equimolar H 2 /CO 2 mixture through a 2-μm-thick MXene membrane at 25 °C and 1 bar. d H 2 /CO 2 separation performance of the MXene membrane compared with state-of-the-art gas separation membranes. The black line indicates the Robeson 2008 upper bound of polymeric membranes for H 2 /CO 2 separation [58] , and the orange dashed line represents the 2017 upper bound of the best current membranes for H 2 /CO 2 separation. Information on the data points is given in Supplementary Table 9 Full size image The 2D structure and tunable physicochemical properties of MXene offer an exciting opportunity to develop a new class of molecular sieving membranes. Considering that more than 30 MXenes are already available [30] and dozens more can be produced, there is certainly plenty of room for improving the performance even further. This work is significant for gas separation, such as H 2 purification, e.g., in methanol reforming process, CO 2 capture for zero-emission fossil fuel power generation, H 2 recovery in ammonia production, etc. Furthermore, it also demonstrates a general concept for 2D membrane design with highly ordered nanochannels enabling fast and precise molecular sieving for mixture separation. Preparation of the MXene membranes The MXene solution was synthesized as follows [29] : one gram of LiF (purchased from Aladdin) was dissolved in 20 ml HCl (6 M, purchased from Sinopharm Chemical Reagent Co., Ltd.,) solution in a 250 ml Teflon beaker. Then, 1 g Ti 3 AlC 2 (purchased from Beijing Jinhezhi Materials Co., Ltd.) was added to the solution with magnetic stirring at 35 °C for 24 h. The resulting product was washed using deionized (DI) water and centrifugated at 3500 rpm several times until the pH of the supernatant >6, and a clay-like sediment was obtained. The sediment was then dispersed in DI water with ultrasonication for 10 min in order to delaminate the MXene flakes. Most of the unexfoliated MXene was removed after centrifugation at 3500 rpm for 1 h. The concentration of the obtained MXene solution was ~0.5 mg ml −1 . The MXene membranes were prepared by filtering a certain amount of the MXene solution on AAO (0.2 µm pore size and a diameter of 35 mm, purchased from Puyuannano Co., Ltd.) substrates using vacuum-assisted filtration (Supplementary Fig. 7 ). All membranes were dried at 70 °C for 24 h and could be easily detached from the substrate (Supplementary Fig. 8 ). During the membrane preparation process, Ar was used to prevent the oxidation. Characterization of the MXene nanosheets and membranes SEM images were obtained using a Hitachi SU8220 device. The SEM elemental mapping analysis was conducted using an EDX (Oxford EDS, with INCA software). TEM images were obtained using a JEOL JEM-2100F microscope with an acceleration voltage of 200 kV. Elemental mapping in TEM was conducted using the Bruker EDS System. The XRD analysis was carried out using a Bruker D8 Advance with filtered Cu-Kα radiation (40 kV and 40 mA, λ = 0.154 nm); the step scan was 0.02°, the 2 θ range was 2–10° or 2–70°, and the step time was 2 s. FTIR was conducted by Bruker VERTEX 33 units in the wavenumber range of 400–4000 cm −1 . The XPS analysis was performed using an ESCALAB 250 spectrometer (Thermo Fisher Scientific) with monochromated Al-Kα radiation (1486.6 eV) under a pressure of 2 × 10 −9 Torr. The AFM images were obtained using a Bruker Multi Mode 8 scanning probe microscope (SPM, VEECO) in tapping mode. The TG measurement was analyzed on a Netzsch STA 449F3 instrument under the flow of N 2 . The adsorption isotherms of H 2 , CO 2 , N 2 , and CH 4 on the MXene membranes were measured using a Micromeritics (ASAP 2460) instrument. The mechanical tests were performed using an Instron-5565 universal testing machine (USA). Gas permeation measurements All the gas permeation measurements were conducted by a homemade membrane module (Supplementary Fig. 20 ). Silicone gaskets were used to avoid the leakage and the direct contact between the stainless-steel module and membranes. The gas transport through the membrane was measured using the constant pressure, variable volume method. A calibrated gas chromatograph (GC, Agilent 7890A) was used to analyze the composition of the permeate gas. During single-gas permeation, a flow rate of 50 ml min −1 gas was used in the feed side of the membrane, and sweep gas with a flow rate of 50 ml min −1 was used to remove the permeated gas on the permeate side. During mixed-gas permeation, a gas mixture with a ratio of 1:1 was applied at the feed side of the MXene membrane, and the total flow rate of the feed gas was maintained at 100 ml min −1 (each gas at 50 ml min −1 ). The gas flow was controlled using mass flow controllers (MFCs). The pressures on both the feed and permeate side were maintained at 1 bar. In most cases, N 2 was used as the sweep gas, except when using a N 2 -containing gas as the feed, then CH 4 was employed as the sweep gas. The gas separation measurements were carried out at different temperatures. The membrane module was packed with heating tape and thermocouple and temperature controller devices were used to control the temperature and heating rate (2 °C min −1 ). Feed gases containing different H 2 concentrations were obtained by adjusting the flow rates of H 2 and CO 2 , which were controlled using the MFCs and calibrated using a bubble flowmeter. Steam (3 vol%) was introduced into the feed gas after passing it through a water tank at room temperature. The different gas pressures at the feed side of the MXene membranes were controlled with a back-pressure valve. All of the gas permeation tests were carried out at least three times. The permeability of each gas was calculated from the following equation [6] : 
    P = 1/Δp×273.15/273.15 + T×P_atm/76×L/A×dv/dt,
 (1) where P is the permeability (1 Barrer = 1 × 10 −10 cm 3 cm cm −2 s −1 cmHg −1 at standard temperature and pressure (STP)); Δ p is the transmembrane pressure (atm); P atm is the atmospheric pressure (atm); T is the temperature (°C); L is the thickness of the membrane (cm); d v/ d t is the volumetric displacement rate in the bubble flowmeter; and A is the effective area of the MXene membrane (1.13 cm 2 ). The selectivity of two components in the single-gas permeation (ideal selectivity) was calculated as follows: 
    α = P_i/P_j,
 (2) where P i and P j are the permeability of each component. The selectivity of two components in the mixed-gas permeation (separation factor) was calculated as follows: 
    α_i/j = y_i/y_j/x_i/x_j,
 (3) where x and y are the volumetric fractions of the corresponding component in the feed and permeate side, respectively [7] . MD simulations Classical MD simulations, which have been proven to be an efficient tool in similar studies [16] , [36] , [38] , were utilized to gain theoretical insight into the gas (e.g., H 2 , He, N 2 , O 2 , CO 2 , and CH 4 ) permeation through the MXene membrane. Two sets of simulations were carried out: one to study the gas molecule permeation through the MXene membrane (Supplementary Fig. 26 , denoted as the flux simulation) [16] , [36] , and another to calculate the gas diffusion coefficient in the MXene subnanometer channels (Supplementary Fig. 25 , denoted as the confined diffusion simulation) [37] , [39] . In the flux simulation, 30 gas molecules were placed in the feed chamber on the left side of (along the z direction) the MXene membrane (Ti 3 C 2 O 2 ) using a structure taken from the literature [40] . The free spacing between the MXene nanosheets was ~3.5 Å (see main text in Fig. 1h ), and 2.4 wt% water as adsorbate was added randomly between the MXene nanosheets, as determined from the experiments (see the experimental TG in Supplementary Fig. 12 ). In order to investigate the effect of the surface functional groups on gas separation, gas permeation through the MXene membranes with another model (Ti 3 C 2 F 2 ) has also been simulated and simulations of gas permeation were conducted through the MXene membrane again (H 2 and CO 2 as examples) (Supplementary Fig. 27 and Supplementary Table 7 ). The MXene nanosheets were modeled by the UFF force field (FF) with QEq charge [41] , [42] , which has been proven to accurately simulate the interactions of gas molecules with nanoporous materials. The water was described using the SPC/E model [43] . The N 2 , O 2 , CO 2 , and CH 4 gas molecules were modeled using the TraPPE FF [44] , [45] , and the united-atom parameters of H 2 and He were taken from other publications [46] , [47] . These FF parameters have been proven to accurately simulate the transport of these five gases in nanoporous materials [39] , [48] , [49] , [50] . In both the flux or diffusion simulation, the system was subjected to a 500-step steepest-descent energy minimization. Then, a 200–300 ns (flux) or 40 ns (diffusion) NVT (constant particle number, volume and temperature) simulation was performed (leap-frog algorithm with a time step of 2 fs). The Nose–Hoover thermostat [51] was employed to maintain a constant simulation temperature of 300 K. The MXene atoms were frozen in the simulations since the nanosheets were rather rigid. The short-range interactions were evaluated using a neighbor list of 10 Å that was updated every ten steps, and the Lennard–Jones interactions were switched off smoothly between 8 and 9 Å. A long-range analytical dispersion correction was applied to the energy to account for the truncation of these interactions [52] . The electrostatic interactions were evaluated using the reaction-field method [53] . During the flux simulation, the gas molecules passed through the membrane to the permeate chamber (along the z direction), driven by the concentration difference, and the flux was calculated as the ratio of the number of gas molecules passing through the membrane to the simulation time. The MXene membrane was 5.5 nm × 5.3 nm in the primary simulation box, and a periodic boundary condition (PBC) was applied to the x – y direction (thus, the MXene membrane was essentially infinite in the x– y direction). The z length of the flux simulation box was 32 nm, and the MXene membrane (length ~5.3 nm) was placed approximately in the middle, leading to the feed chamber of ~12.6 nm long, and the permeate chamber of ~14.1 nm long. Considering the lateral size of the MXene flakes in the experiments was 1–2 μm, confined diffusion simulations were also performed, in which six gas molecules (H 2 , He, N 2 , O 2 , CO 2 , and CH 4 ) diffused between two MXene nanosheets (without the presence of a feed chamber or permeate chamber). These two MXene nanosheets with a free spacing of 0.35 nm were essentially infinite since the PBC was applied during the MD simulations, although they were 5.5 nm × 5.3 nm in the primary simulation box. During the confined diffusion simulation, the gas molecules diffused in two neighboring MXene nanosheets (a confined subnanochannel), and for each gas, a 40 ns NVT calculation was carried out and using the Einstein relation, 
    D = lim_t→∞1/6t( 1/N∑_N^k = 1| r_k(t) - r_k(0)|^2),
 (4) where r k ( t ) is the position of the k th molecule at time t and N is the number of molecules. All MD simulations in this work were performed using the GROMACS 4.6.7 package [54] , [55] , while the simulation trajectories were analyzed using the GROMACS utilities and home-written codes. The interaction energies of the gas molecules with the MXene nanosheets were calculated from the diffusion simulation trajectories. Figures of the simulated systems were produced using VMD software [56] . Each flux simulation (200 ns for the single-gas permeation of H 2 , N 2 , O 2 , CO 2 with 30 gas molecules in the simulation system; 300 ns for the mixed-gas permeation of H 2 + N 2 and H 2 + CO 2 with 60 gas molecules in the simulation system, 30 for each gas species) was repeated four times, and the averaged flux was reported. The flux simulations of the single-gas permeation (in which only one gas was used, e.g., H 2 , N 2 , O 2 , or CO 2 ) were also performed with a very long permeate cell (~60 nm, denoted as the long-box simulations) to mimic the experiments more closely. The long-box simulations yielded very similar results compared to the normal-box simulation with a 14.1 nm long permeate cell (except for H 2 in which the flux changed a little from 0.75 to 0.90 molecule ns −1 ). Thus, the flux simulation refers to the normal size box ( z length of the box = 32 nm, permeate cell length = 12.6 nm, permeate cell length = 14.1 nm, main text Fig. 2d and Supplementary Fig. 26 ) in this work unless otherwise specified. Each diffusion simulation (H 2 , He, N 2 , O 2 , CO 2 , and CH 4 ) was 40 ns long. Thus, the total simulation time was 5 μs or more (4 × 3 × 200 ns + 4 × 2 × 300 ns + 5 × 40 ns = 5 μs). See our previous publications for further simulation details [57] . Data availability The data sets generated and analyzed during the current study are available from the corresponding authors on reasonable request.